Neolithic mitochondrial haplogroup H genomes and the genetic origins of Europeans Haplogroup H dominates present-day Western European mitochondrial DNA variability (>40%), yet was less common (~19%) among Early Neolithic farmers (~5450 BC) and virtually absent in Mesolithic hunter-gatherers. Here we investigate this major component of the maternal population history of modern Europeans and sequence 39 complete haplogroup H mitochondrial genomes from ancient human remains. We then compare this ‘real-time’ genetic data with cultural changes taking place between the Early Neolithic (~5450 BC) and Bronze Age (~2200 BC) in Central Europe. Our results reveal that the current diversity and distribution of haplogroup H were largely established by the Mid Neolithic (~4000 BC), but with substantial genetic contributions from subsequent pan-European cultures such as the Bell Beakers expanding out of Iberia in the Late Neolithic (~2800 BC). Dated haplogroup H genomes allow us to reconstruct the recent evolutionary history of haplogroup H and reveal a mutation rate 45% higher than current estimates for human mitochondria. A key unanswered issue in human prehistory is the extent to which cultural change identifiable in the archaeological record can be ascribed to the movements of people, as opposed to the movements of just their ideas and artefacts. The Central European archaeological record identifies a succession of profound cultural and economic changes between the last hunter-gatherers of the Mesolithic and the first farmers of the Early Neolithic (ENE), through to the socially stratified chiefdoms of the Early Bronze Age [1] , [2] , [3] . The exact nature and genetic context of the transformative changes that took place over these four millennia remain unclear [4] , [5] , although current genetic patterns of mitochondrial DNA (mtDNA) haplogroup (hg) distribution suggest a complex series of events in European prehistory [4] , [5] , [6] , [7] , [8] , [9] and hint at multiple inputs from outside Central Europe [4] , [10] , [11] . Phylogeographic studies suggest that mt hg H arrived in Europe from the Near East before the Last Glacial Maximum (22,000 BP), and survived in glacial refugia in Southwest Europe before undergoing a post-glacial re-expansion [4] , [12] . Haplogroup H now accounts for over 40% of mtDNA variation in anatomically modern humans across much of Western Eurasia, with declining frequencies south and east to ~10–30% in the Near East and Caucasus [10] . However, it remains uncertain when and how H became the dominant European hg. Traditional approaches (including ancient DNA studies) have been unable to resolve either the phylogeny or phylogeographic distribution of H sub-haplogroups (sub-hgs) [6] , however, they have generally relied on sequencing only 300–400 bp of the mt D-loop or control region [10] , [13] . A number of studies based on complete 16.6 kb human mt genomes have revealed a complex evolutionary history for hg H (for example, refs 12 , 14 , 15 , 16 , 17 , 18 , with phylogenetic analyses recognizing 87 H sub-hgs [19] ). These complete mt genomes revealed that 71% of hg H polymorphic diversity is located outside the D-loop, in the coding region [20] and, as a result, this diversity has not yet been exploited at the population genetics level. To investigate the relationship between the European genetic and archaeological records, we sequenced whole hg H mt genomes from skeletal remains directly assigned to distinct Central European archaeological cultures. Owing to its excellently preserved human skeletal remains, forming a continuous record across a series of archaeological cultures since Palaeolithic times, the Mittelelbe-Saale region of Saxony-Anhalt (Germany) provided a unique opportunity to address this issue. 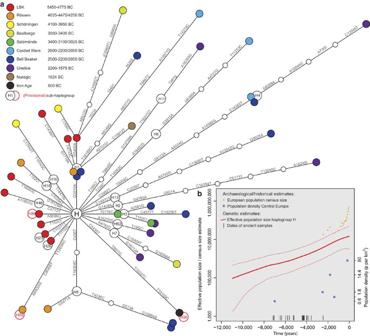Figure 1: Mitochondrial haplogroup H sequence evolution. (a) Phylogenetic network of 39 prehistoric mitochondrial genomes sorted into two temporal groupings: Early Neolithic (left) and Mid-to-Late Neolithic (right). Node colours represent archaeological cultures. (b) A Bayesian skyride plot of 200 representative present-day and 39 ancient hg H mt genomes (the thick red line denotes the posterior median, thinner flanking lines denote the 95% credibility interval; note the logarithmic scale of theyaxis). Prehistoric samples (18 radiocarbon and 21 mean archaeological dates) served as internal calibration points (black bars). For comparison, census size estimates for the European population are shown as orange dots. Population density estimates from the archaeological record for key periods in Central Europe are plotted as blue squares in chronological order: LBK, Iron Age, Roman period, Merovingian and Pre-industrial modern times (yaxis on the right)28. We analysed a time transect spanning the >3,500 years of the Central European Neolithic period ( Table 1 , Supplementary Table S1 ), from the first farmers of the ENE linear pottery culture (LBK, 5450–4775 BC), through the subsequent Rössen (4625–4250 BC), Schöningen (4100–3950 BC), Baalberge (3950–3400 BC) and Salzmünde (3400–3025 BC) cultures. These were followed by two of the first pan-European Late Neolithic (LNE) cultural complexes, the Corded Ware (CWC, 2800–2050 BC) and Bell Beaker (BBC, 2500–2050 BC) cultures, before the emergence of the Early Bronze Age with the Unetice culture (2200–1575 BC). We chose to focus on hg H because of its recent dramatic rise in frequency to become the dominant hg in Europe, because of its presence in all Neolithic cultures in the Mittelelbe-Saale region, and the potential it provided to explore detailed genetic structure on a sub-hg level. Overall, our results suggest that the broad foundations of the Central European mtDNA pool, here approximated via hg H, were formed during the Neolithic rather than the post-glacial period. Table 1 Summary of genotyping data against the Reconstructed Sapiens Reference Sequence (RSRS). Full size table Sequence and network analyses From a collection of over 400 European prehistoric human archaeological remains we selected 37 Mittelelbe-Saale individuals, as well as two samples from Italy ( Supplementary Table S1 ), previously assigned to hg H by simplex and multiplex PCR [7] . Work was independently replicated for two samples per individual ( Supplementary Methods ). We designed and optimised a hybridisation-based DNA-capture system to sequence complete mt genomes on the Affymetrix MitoChip v2.0 (ref. 21 ) ( Supplementary Methods , Supplementary Fig. S1,S2 , and Supplementary Tables S2-S3 ) via immortalised libraries prepared from the highly damaged and degraded endogenous DNA recovered from archaeological remains [22] , [23] . Six of the 39 target-enriched libraries were also analysed via a single-molecule, real-time (SMRT [24] ) Pacific Biosciences RS sequencing platform ( Supplementary Table S4 , Supplementary Data set). In addition, 35/391 (9%) of all SNPs identified via the MitoChip were independently confirmed by direct PCR and Sanger sequencing ( Supplementary Methods , Supplementary Tables S5 and S6 ). Mt genomes from all 39 individuals were unambiguously assignable to individual sub-hgs of hg H [20] , confirming that a single human was typed in each case ( Table 1 ). The mt hypervariable region I sequences matched those previously determined for each individual. The ancient hg H mt genomes were highly diverse, with 34 distinct haplotypes attributed to 20 major sub-hgs (gene diversity H=0.997 +/− 0.0071; nucleotide diversity 0.000421 +/− 0.000225), including three novel lineages (provisionally named H88–H90). Phylogenetic network analysis of these ancient mt genomes reveals evidence of dynamic changes in the composition of H sub-hgs over the ~3,500-year time transect ( Fig. 1 ). Importantly, sequences from older samples (and cultures) tend to represent basal lineages, only one to three mutations away from the ancestral root of hg H, while younger samples (after ~4000 BC) largely comprise more derived haplotypes appearing on longer branches. This temporal relationship provides further support for the authenticity of the ancient mt genomes. Figure 1: Mitochondrial haplogroup H sequence evolution. ( a ) Phylogenetic network of 39 prehistoric mitochondrial genomes sorted into two temporal groupings: Early Neolithic (left) and Mid-to-Late Neolithic (right). Node colours represent archaeological cultures. ( b ) A Bayesian skyride plot of 200 representative present-day and 39 ancient hg H mt genomes (the thick red line denotes the posterior median, thinner flanking lines denote the 95% credibility interval; note the logarithmic scale of the y axis). Prehistoric samples (18 radiocarbon and 21 mean archaeological dates) served as internal calibration points (black bars). For comparison, census size estimates for the European population are shown as orange dots. Population density estimates from the archaeological record for key periods in Central Europe are plotted as blue squares in chronological order: LBK, Iron Age, Roman period, Merovingian and Pre-industrial modern times ( y axis on the right) [28] . Full size image Network analysis ( Fig. 1 ) reveals pronounced differences in the composition of sub-hgs between the ENE cultures (LBK, Rössen, Schöningen), and those of the Mid Neolithic (MNE)/LNE to Early Bronze Age (Baalberge, Salzmünde, Corded Ware, Bell Beaker, Unetice). ENE (and in particular LBK) mt genomes are either rare today (H16, H23 and H26), extinct or have not yet been observed in present-day populations (H46b, H88 and H89). In sharp contrast, most of the later H sub-hgs are more common in present-day European populations (for example, hg H3, H4, H6, H7, H11 and H13) [12] , [14] , [15] , [16] . Of the 39 haplotypes detected, only three (within the common, basal, sub-hg H1) were shared between ENE and MNE/LNE cultures. As the observed gene diversity is high, we might expect the number of shared haplotypes within and between cultures to be low. However, as the MNE/LNE haplotypes are on different sub-hg branches from the ENE haplotypes, these patterns combined show minimal local genetic continuity over this time period ( Table 1 ). 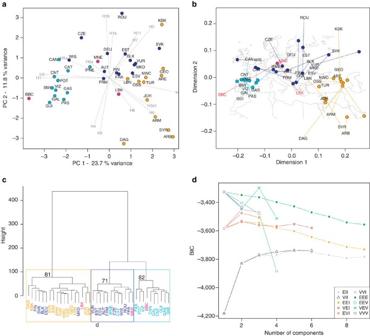Figure 2: Population affinities of select Neolithic cultures. (a) PCA biplot based on the frequencies of 15 hg H sub-haplogroups (component loadings) from 37 present-day Western Eurasian and three ancient populations (light blue: Western Europe; dark blue: Central and Eastern Europe; orange; Near East, Caucasus and Anatolia; and pink: ancient samples). Populations are abbreviated as follows: GAL, Galicia; CNT, Cantabria; CAT, Catalonia; GAS, Galicia/Asturia; CAN, Cantabria2; POT, Potes; PAS, Pasiegos; VIZ, Vizcaya; GUI, Guipuzcoa; BMI, Basques; IPNE, Iberian Peninsula Northeast; TUR, Turkey; ARM, Armenia; GEO, Georgia; NWC, Northwest Caucasus; DAG, Dagestan; OSS, Ossetia; SYR, Syria; LBN, Lebanon; JOR, Jordan; ARB, Arabian Peninsula; ARE, Arabian Peninsula2; KBK, Karachay-Balkaria; MKD, Macedonia; VUR, Volga-Ural region; FIN, Finland; EST, Estonia; ESV, Eastern Slavs; SVK, Slovakia; FRA, France; BLK, Balkans; DEU, Germany; AUT, Austria, ROU, Romania; FRM, France Normandy; WIS, Western Isles; CZE, Czech Republic; LBK, Linear pottery culture; BBC, Bell Beaker culture; MNE, Middle Neolithic. (b) Procrustes analyses of geographic coordinates and PCA scores of the same data set (similarity scoret0=0.733,P<10−6, 100,000 permutations). (c) Ward clustering dendrogram of the three ancient groups and present-day populations (colour code as above and p values in % of approximately unbiased bootstrapping for the following three main clusters). (d) Results of the model-based test to identify the number of clusters by the model with the highest support (highest Bayes Information criterion (BIC); VEV=multivariate mixture model (ellipsoidal, equal shape)). Genetic distances To further examine these apparent temporal shifts in sub-hg distribution, we tested whether hg H individuals represent different meta-populations by pooling them into different cultural and/or temporal groups of ENE versus LNE ( Table 2 , Supplementary Table S7 ). When pooled in four groups (ENE, MNE, LNE and Bronze Age), pairwise population comparisons via F ST values based on sequence data showed that genetic distances increased with time over the duration of the Neolithic, reaching a significant value ( F ST =0.08722; P =0.00386+/−0.0006) between the ENE and the early Bronze Age ( Table 2 ). This suggests a transformation of hg H diversity during the Neolithic period. This effect was less apparent (non-significant F ST values) when samples from various sites were pooled in larger temporal groups ( Table 2 ). However, non-parametric multivariate analysis of variance (NP-MANOVA, P =0.0072) also confirmed a significant difference between pooled groups of ENE and LNE individuals when comparisons were based on the presence or absence of sub-hgs ( Table 2 ). Table 2 Population pairwise and linearised Slatkin’s F ST s and NP-MANOVA tests. Full size table Genetic affinities To examine potential geographic origins for Neolithic cultures ( Supplementary Table S1 ) and to assess their contribution to present-day Central European mtDNA diversity, we used principal component analysis (PCA) to investigate genetic affinities between three ancient culturally/temporally pooled groups (LBK, MNE and BBC) and 37 present-day Western Eurasian populations ( Supplementary Table S8 ). PCA of the frequencies of the 15 most common H sub-hgs showed that the present-day populations form three significantly supported geographic clusters (a grouping which was also supported using NP-MANOVA, P <0.0001; Table 2 : (i) Iberia in the west; (ii) the Caucasus, the Near East and Anatolia; and (iii) Central and Eastern Europe from the Urals to France ( Fig. 2a ). This particular number of clusters was also the best supported in a model-based test on sub-hg H frequencies followed by Ward clustering ( Fig. 2c ). We also used Procrustes analysis to quantify the relationship between hg H substructure and the geographic locations of both the present-day Western Eurasian and the Mittelelbe-Saale ancient populations. For this analysis, we superimposed the PCA coordinates on the geographic map of the present-day and ancient sampling locations. We found a striking resemblance between the genetic and geographic maps, with a highly significant Procrustes similarity score ( t 0 =0.733) obtained for the comparison ( P <10 −6 ; 100,000 permutations). The analysis supported a clustering of the transformed genetic data from present-day populations into the three major groups described above ( Fig. 2b ). In contrast, Procrustes analysis clearly showed that the genetic data for LBK and BBC samples were not related to their geographic location. Although all three ancient groups were sampled from the same Central European location only the MNE group genetically resembles present-day populations from this region. Figure 2: Population affinities of select Neolithic cultures. ( a ) PCA biplot based on the frequencies of 15 hg H sub-haplogroups (component loadings) from 37 present-day Western Eurasian and three ancient populations (light blue: Western Europe; dark blue: Central and Eastern Europe; orange; Near East, Caucasus and Anatolia; and pink: ancient samples). Populations are abbreviated as follows: GAL, Galicia; CNT, Cantabria; CAT, Catalonia; GAS, Galicia/Asturia; CAN, Cantabria2; POT, Potes; PAS, Pasiegos; VIZ, Vizcaya; GUI, Guipuzcoa; BMI, Basques; IPNE, Iberian Peninsula Northeast; TUR, Turkey; ARM, Armenia; GEO, Georgia; NWC, Northwest Caucasus; DAG, Dagestan; OSS, Ossetia; SYR, Syria; LBN, Lebanon; JOR, Jordan; ARB, Arabian Peninsula; ARE, Arabian Peninsula2; KBK, Karachay-Balkaria; MKD, Macedonia; VUR, Volga-Ural region; FIN, Finland; EST, Estonia; ESV, Eastern Slavs; SVK, Slovakia; FRA, France; BLK, Balkans; DEU, Germany; AUT, Austria, ROU, Romania; FRM, France Normandy; WIS, Western Isles; CZE, Czech Republic; LBK, Linear pottery culture; BBC, Bell Beaker culture; MNE, Middle Neolithic. ( b ) Procrustes analyses of geographic coordinates and PCA scores of the same data set (similarity score t 0 =0.733, P <10 −6 , 100,000 permutations). ( c ) Ward clustering dendrogram of the three ancient groups and present-day populations (colour code as above and p values in % of approximately unbiased bootstrapping for the following three main clusters). ( d ) Results of the model-based test to identify the number of clusters by the model with the highest support (highest Bayes Information criterion (BIC); VEV=multivariate mixture model (ellipsoidal, equal shape)). Full size image The combined set of analyses (PCA, Procrustes and Ward clustering) revealed that Mittelelbe-Saale’s earliest farmers (LBK; n =9) cluster with present-day Caucasus, Near Eastern and Anatolian populations, as previously noted [7] . In contrast, individuals from the successor series of regional post-LBK (and MNE) Rössen, Schöningen, Baalberge and Salzmünde cultures (ca. 4625–3025 BC, MNE; n =10) cluster with present-day Central European populations ( Fig. 2 ). Mitochondrial genomes from BBC individuals in Mittelelbe-Saale (BBC; n =7) display close genetic affinities to present-day Iberian populations ( Fig. 2 ). The component loadings of the PCA biplot indicate that this is largely based on high frequencies of sub-hgs H1 and H3, which are thought to have spread from a glacial Iberian refugium [13] and which have also been reported from ancient Neolithic sites from France and Spain [8] , [25] . Other LNE samples add further to the genetic complexity. Individuals from the CWC (2800–2200 BC), which has archaeological associations towards North-Eastern Europe, produced two distinct mt genomes (H1_TBD and H6a1a), which have not been found in their contemporaneous Bell Beaker neighbours, nor in preceding Central European cultures. Similarly, data from the subsequent Early Bronze Age Unetice culture revealed haplotypes with genetic affinities to both the East (sub-hg H2a, H7 and H11) and the West (sub-hg H3 and H4), based on frequency distributions of these sub-hgs in present-day populations [13] . We also included two individuals from outside Central Europe (Sardinia and South Tyrol) and from different time periods (Nuragic Bronze Age and Iron Age, respectively) to further investigate genetic diversity within hg H and to test the power of resolution of complete mt genomes. Both individuals had mt genomes that are not found in samples from the Mittelelbe-Saale region. The Iron Age sample from South Tyrol produced another new sub-hg (provisional H90) and the Bronze Age individual from Sardinia a new H1 haplotype (H1aw1). Reconstructing the demographic history of mtDNA hg H It has previously proved difficult to use present-day data alone to determine when hg H became the predominant hg in Europe, as archaeogenetic and palaeodemographic reconstructions have very large uncertainties [4] , [26] . However, as our 39-dated ancient mt genome sequences provide precise temporal calibration points, we performed a Bayesian skyride analysis with 200 random present-day mt genome sequences to reconstruct the lineage history of hg H through time (with the caveat of assuming a continuous and panmictic population). The resulting skyride plot ( Fig. 1b ) is the first real-time estimation of the European hg H population size (and consequently its contribution to Europe’s effective population size and demographic history) with a broad temporal coverage over ~3,500 years of the Neolithic period in Central Europe (5500–2000 BC). Hg H shows a consistent and strong exponential growth over the entire course of the Neolithic. The estimated population size tracks the European census size [27] and population density estimates from archaeological sites [28] in the Late Holocene, but also provides detailed estimates for prehistoric times for which data points remain very scarce ( Fig. 1b ). Another major advantage of the temporal calibration points provided by ancient hg H mt genomes is that the data allow a relatively precise estimate of the evolutionary substitution rate for human mtDNA. The temporal dependency of evolutionary rates predicts that rate estimates measured over short timespans will be considerably higher than those using deep fossil calibrations, such as the human/chimpanzee split at ~6 million years [29] . The rate calibrated by the Neolithic and Bronze Age sequences is 2.4 × 10 −8 substitutions per site per year (1.7–3.2 × 10 −8 ; 95% high posterior density) for the entire mt genome, which is 1.45 × (44.5%) higher than current estimates based on the traditional human/chimp split (for example, 1.66 × 10 −8 for the entire mt genome [30] and 1.26 × 10 −8 for the coding region [31] ). Consequently, the calibrated ‘Neolithic’ rate infers a considerably younger coalescence date for hg H (10.9–19.1 kya) than those previously reported (19.2–21.4 kya for HVSI [10] , 15.7–22.5 kya for the mt coding region [31] or 14.7–22.6 kya when corrected for purifying selection [30] ). Despite recent successes in sequencing portions of nuclear genomes from Meso- and Neolithic samples [11] , [32] , [33] , mtDNA remains the most widely studied and best described marker in population genetics. Although its interpretation is limited to the matrilineal genetic history [4] , [13] , [19] , this can be an important socio-cultural and demographic signal additional to that gained from autosomal loci [34] , [35] . Our results clearly demonstrate that high-resolution full mt genome-typing, combined with the ability to analyse large numbers of individuals from multiple cultural layers, can provide highly resolved temporal views that are not yet practical with nuclear DNA studies. The phylogenetic network analysis of our chronological hg H mt genome data set ( Fig. 1a ) provides the first detailed real-time view of mutations in human mtDNA. It has enabled the direct observation of the mutation rate over thousands of years and revealed a distinct temporal distribution pattern of hg H diversity. Although a temporal pattern could be expected in an expanding population with stable/increasing hg H frequencies ( Fig. 1b , Supplementary Fig. S3 ), ENE and MNE/LNE/Bronze Age samples clearly show a mutually exclusive sub-hg distribution with the exception of sub-hg H1, which is the most common and basal sub-hg within H [14] , [15] , [16] . Under an assumption of genetic continuity, we would expect MNE/LNE and Bronze Age individuals to be on the same sub-hg branches as ENE individuals. Instead, ENE mt genomes are generally either rare today [19] or have not yet been observed in present-day populations, possibly owing to subsequent extinction of these lineages. In contrast, most MNE/LNE and Bronze Age sub-hgs are still common today. This suggests that individuals from the ENE made a marginal contribution to LNE and present-day hg H diversity. Although the relatively small sample numbers from each time period limit detailed analyses of the causes of the distribution shifts, we interpret this phylogenetic pattern as a genetic discontinuity between Early and subsequent Neolithic cultures in Europe, potentially mirroring genetic structure in Neolithic European populations. Genetic drift could also have played a role in generating discrepant hg distributions over time and space. However, if drift was the sole cause we would expect a random distribution across all sub-hgs rather than a clear distinction between ENE and MNE/LNE/Bronze Age mt genomes. Our genetic distance data also indicate minimal local genetic continuity between the ENE and the MNE/LNE in Central Europe ( Fig. 1 ; Table 1 ), again suggesting that ENE lineages were largely superseded during the MNE/LNE (~4100–2200 BC) in a previously unrecognised major genetic transition. This pronounced genetic changeover between ENE and MNE/LNE cultures is comparable to other known major genetic transition, thus far revealed by ancient DNA and coalescent simulations (between indigenous European hunter-gatherers and incoming early farmers from the Near East during the initial Meso-Neolithic transition from ~7500 BC in Central Europe) [6] , [7] . When compared with hg H diversity in present-day Central Europe [14] , [15] , [18] , [36] , the network in Fig. 1 suggests that much of the present-day diversity can be attributed to the incorporation of new lineages in the MNE/LNE and emerging Bronze Age (from 2200 BC). The LNE in particular is known to have been a period of profound cultural and economic change [37] , with newly emerging pan-European cultures such as the Bell Beaker phenomenon in Western Europe and the Corded Ware culture in north-eastern Europe. It therefore seems likely that these pan-European cultures were associated with the introduction of lineages from outside Central Europe. Fortunately, the ranges of both these groups overlapped in the Mittelelbe-Saale sample area ( Supplementary Methods ), allowing this possibility to be further investigated. Our data on genetic affinities (PCA, Procrustes and Ward clustering) revealed that Mittelelbe-Saale’s earliest farmers (LBK; n =9) cluster with present-day Caucasus, Near Eastern, and Anatolian populations. These findings are consistent with a highly detailed archaeological record tracing the temporal and spatial spread of agriculture into Central Europe; beginning initially in Anatolia and the Near East, where farming originated ~12,000 years ago 7 . Our observation that individuals from the successor series of regional post-LBK and MNE cultures (Rössen, Schöningen, Baalberge and Salzmünde) cluster with present-day Central European populations could be explained by a loss of lineages from the ENE LBK period during a short phase of population decline in the centuries after 5000 BC (as proposed in some archaeological models) [38] . However, our results suggest that mtDNA H sub-hg diversity established during the MNE is still present in Central European populations today. This is consistent with independent archaeological evidence of a phase of more localised cultural development during the MNE period, potentially involving influences from contemporaneous MNE cultures outside Mittelelbe-Saale, which (perhaps in concert with LBK population decline) could have resulted in a replacement of most ENE H sub-hgs. Together, the genetic and archaeological evidence highlight the complexities of both the formative and consolidation phases in Central Europe. From around 2800 BC, the LNE Bell Beaker culture emerged from the Iberian Peninsula to form one of the first pan-European archaeological complexes. This cultural phenomenon is recognised by a distinctive package of rich grave goods including the eponymous bell-shaped ceramic beakers. The genetic affinities between Central Europe’s Bell Beakers and present-day Iberian populations ( Fig. 2 ) is striking and throws fresh light on long-disputed archaeological models [3] . We suggest these data indicate a considerable genetic influx from the West during the LNE. These far-Western genetic affinities of Mittelelbe-Saale’s Bell Beaker folk may also have intriguing linguistic implications, as the archaeologically-identified eastward movement of the Bell Beaker culture has recently been linked to the initial spread of the Celtic language family across Western Europe [39] . This hypothesis suggests that early members of the Celtic language family (for example, Tartessian) [40] initially developed from Indo-European precursors in Iberia and subsequently spread throughout the Atlantic Zone; before a period of rapid mobility, reflected by the Beaker phenomenon, carried Celtic languages across much of Western Europe. This idea not only challenges traditional views of a linguistic spread of Celtic westwards from Central Europe during the Iron Age, but also implies that Indo-European languages arrived in Western Europe substantially earlier, presumably with the arrival of farming from the Near East [41] . Other LNE population movements appear to have added further genetic complexity, as exemplified by the CWC (2800–2200 BC), which preceded the Bell Beaker culture in Mittelelbe-Saale and has archaeological associations with North-Eastern Europe. A genetic affinity to eastern populations is consistent with two distinct CWC mt genomes (H1_TBD and H6a1a) not identified in either their contemporaneous Bell Beaker neighbours or in preceding Central European cultures. The subsequent Early Bronze Age Unetice culture, associated with emerging metallurgy and increasingly stratified societies [37] , [42] , marks a consolidation of social and cultural systems in Mittelelbe-Saale that were established during the LNE by the two pan-European Bell Beaker and CWCs. The Unetice culture appears contemporaneously with the last Neolithic horizon (~2200 BC) in areas where elements of both the Bell Beaker and CWCs are present, sometimes overlapping at the same sites. It is therefore not surprising that individuals ascribed to the newly emerging Unetice culture carry mt genomes with both Western (sub-hgs H3 and H4) and Eastern (sub-hgs H2a, H7 and H11) associations. The demographic reconstruction, which is based on direct calibration points, has major implications for understanding post-glacial human history in Europe. Our new estimate is incompatible with traditional views that the majority of present-day hg H lineages were carried into Central, Northern and Eastern Europe via a post-glacial human population expansion before the Holocene (12 kya) [13] . Our data complement a recent study, based on present-day mt genomes, which describes a pronounced population increase at ~7000 BC (interpreted as a Neolithic expansion into Europe), but followed by a slow population growth until the present day [26] . By including ancient DNA data from across the critical time points in question, our skyride plot corrects for missing temporal data and suggests substantial growth of hg H from the beginning of the Neolithic and continuing throughout the entire Neolithic period. This emphasizes the role of farming practices and cultural developments in the demographic expansions inferred in subsequent time periods, which have not yet been explored genetically. Although an expansion of hg H could in principle be compatible with a post-glacial resettling of Northern and Central Europe from southwestern refugia [12] , [16] (as indicated by our population skyride and PCA plots), we instead propose that the rise of hg H to become the predominant mtDNA branch in Europe was mediated by subsequent demographic events during the Neolithic, as shown by a general increase in hg H frequency and strong population growth during this period ( Fig. 1b ). Support for this position comes from data suggesting that hg H was virtually absent among Central and Northern European hunter-gatherers [6] , [43] and formed only 19% in LBK individuals, most likely introduced from Southeast Europe and/or the Near East [7] . In our updated data set from Mittelelbe-Saale, hg H appears to have been established by the LBK period and increased in frequency after 4000 BC ( Supplementary Fig. S3 ). Interestingly, MNE/LNE cultures with cultural associations to the North and Northeast, such as the Bernburg and CWCs, show reduced hg H frequencies and hg H only moved northwards into southern Scandinavia during the Neolithisation of Northern Europe around the Middle Neolithic, as exemplified by individuals from the Funnel Beaker Culture [11] , [43] . However, hg H appears to have been generally more frequent in prehistoric Western Europe: at 20% from a Middle Neolithic (3030–2890 calBC) site in France [9] ; at ~25% from Iberian (Epi-)Cardial Neolithic samples [8] , [25] ; at 36% from a Neolithic site in Catalonia [44] ; and at 44% from Neolithic sites from the Basque Country and Navarre [45] . Importantly, a recent study on Iberian hunter-gatherers revealed the presence of hg H there in Mesolithic times [45] . In Mittelelbe-Saale, the Bell Beaker samples signpost a significant increase in hg H frequency (the 95% confidence intervals do not overlap with earlier LBK and Schöningen Neolithic cultures; Supplementary Fig. S3 ). In conclusion, the Western European Neolithic and the widespread pan-European Bell Beaker phenomenon appear to be important factors in driving the spread of H sub-hgs throughout large parts of Western Europe. In particular, high proportions of sub-hgs H1 and H3 seem to have made substantial contributions to the hg H diversity that exists in Western and Central Europe today [16] . Having reached significant levels, and assuming a generally higher rate of population growth in southern and western Europe in post-Neolithic times [27] , these Neolithic processes appear to have been the major factor in hg H becoming the predominant European mtDNA hg. Overall, our results suggest that the broad foundations of the Central European mtDNA pool, here approximated via hg H, were formed during the Neolithic rather than the post-glacial period. ENE hg H mt lineages brought in from the Near East by Central Europe’s first farmers do not appear to have contributed significantly to present-day Central Europe’s hg H diversity, instead being largely superseded during the MNE and LNE (with the process starting around 4000 BC), after which there appears to have been substantial genetic continuity to the present-day in Central Europe. These developments have been revealed by comparative full mt genome sequencing and would have remained obscure using standard HVS I data. In conclusion, demographic changes across the MNE, followed by the widespread Bell Beaker cultural phenomenon, are likely to have been the key factors in the expansion of hg H across Western Europe and the eventual rise of hg H to become the predominant mtDNA hg. However, LNE Corded Ware and Early Bronze Age data suggest a complex series of additional genetic contributions, which require further investigation. Ancient DNA analyses DNA was extracted from two independent samples for each individual ( Supplementary Methods ). HVS I was amplified using a minimum of four short overlapping primer pairs, following established protocols and authentication criteria as described previously [7] , [46] . Multiplex SNP typing of 22 hg informative SNPs (GenoCoRe22) was carried out using a SNaPshot-based protocol as described previously [7] . Ancient DNA Library preparation Ancient DNA extract polishing, phosphorylation, adaptor ligation and polymerase ‘fill-in’ reactions were used sequentially to create fully double-stranded adaptor-tagged aDNA libraries ( Fig. 3 ). Following every step, DNA was purified using MinElute spin columns (Qiagen) as per the manufacturer’s instructions. PCR amplification reactions were then performed to create ‘primary’ DNA libraries, ready for DNA-capture hybridisation steps, and amplification products were sized and quantified ( Supplementary Methods ). 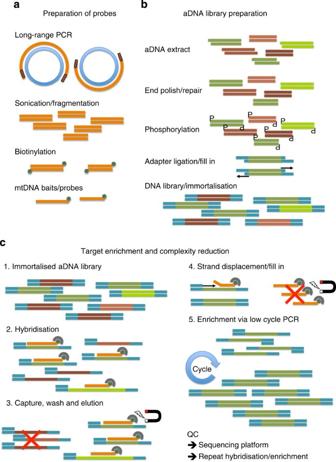Figure 3: Schematic representation of experimental steps. (a) Probe DNA was prepared by amplifying a complete mitochondrial genome in two overlapping fragments by long-range PCR, followed by DNA fragmentation and biotinylation to form mtDNA ‘baits’ for targeted hybridisation. (b) Ancient DNA was enzymatically blunt-ended and phosphorylated, ligated to custom library adaptors, followed by polymerase ‘fill-in’ to create ‘immortalised’ double-stranded DNA libraries. (c) Hybridisation-based DNA-capture using biotinylated probe bound to Streptavidin magnetic beads; following stringency washes, captured library constructs enriched in mtDNA sequences are eluted from the beads/probe via a novel polymerase strand-displacement reaction followed by PCR library reamplification. These steps can be carried out iteratively to maximise mtDNA content in enriched libraries (seeSupplementary Methodsfor full details). Figure 3: Schematic representation of experimental steps. ( a ) Probe DNA was prepared by amplifying a complete mitochondrial genome in two overlapping fragments by long-range PCR, followed by DNA fragmentation and biotinylation to form mtDNA ‘baits’ for targeted hybridisation. ( b ) Ancient DNA was enzymatically blunt-ended and phosphorylated, ligated to custom library adaptors, followed by polymerase ‘fill-in’ to create ‘immortalised’ double-stranded DNA libraries. ( c ) Hybridisation-based DNA-capture using biotinylated probe bound to Streptavidin magnetic beads; following stringency washes, captured library constructs enriched in mtDNA sequences are eluted from the beads/probe via a novel polymerase strand-displacement reaction followed by PCR library reamplification. These steps can be carried out iteratively to maximise mtDNA content in enriched libraries (see Supplementary Methods for full details). Full size image Hybridisation-based enrichment of human mtDNA The basic conceptual design for the hybridisation of tracer DNA (aDNA library) to biotinylated driver DNA sequences (human mt probe) was previously described [47] and the overall scheme is outlined in Fig. 3 . The two library-specific PCR primers were included as part of the hybridisation mix as blocking oligonucleotides to minimise unwanted hybridisation between the adaptor-tagged flanking regions of otherwise unrelated single-stranded library DNA molecules [48] . A key innovation of this methodology was the use of a DNA polymerase with strand-displacing activity after post-hybridisation stringency washes. This allowed primer extension from the bound library (blocking) primers to disrupt the double-stranded region of stable hybridisation between human mt probe DNA sequences and single-stranded library DNA molecules that had inserts with complementary sequences. These mtDNA-enriched library DNA molecules captured in the hybridisation step could thereby be cleanly separated from biotinylated probe molecules, which remained bound to magnetic Streptavidin beads. PCR reamplification reactions from the mt-enriched library DNA molecules comprised the ‘first enrichment’ DNA libraries. In general, we used three cycles of hybridisation/enrichment/reamplification to produce DNA libraries highly enriched for short endogenous mtDNA sequence fragments ready for genotyping ( Supplementary Methods ). Affymetrix Mitochip v2.0 array typing and Pacific Biosciences SMRT sequencing MtDNA-enriched libraries underwent biotin labelling using terminal deoxynucleotidyl transferase (TdT) as per the Affymetrix GeneChip Whole-Transcript Sense Target Labelling Assay Manual (P/N 701880, rev. 4). Biotin-labelled DNA libraries were hybridised to Affymetrix GeneChip Human mt Resequencing 2.0 Arrays for 17 h at 49 °C. Arrays were washed, stained and scanned as per the GeneChip CustomSeq Resequencing Array Protocol (P/N 701231, rev. 5). Affymetrix GeneChip Command Console software (v3.2) was used to generate CEL files, which were then analysed using GeneChip Sequence Analysis Software (GSEQ v4.1, Affymetrix) and validated using the software Geneious [49] ( Supplementary Fig. S1,S2 , Supplementary Tables S2,S3 ). Six of the mt-enriched DNA libraries were also converted to SMRTbell template libraries for sequencing on a Pacific Biosciences RS platform ( Supplementary Methods ). Network analyses A median joining network of all ancient hg H mt genomes ( Fig. 1a ) was constructed manually using the most up-to-date version of the mt phylogenetic tree (PhyloTree.org, mtDNA tree Build 14) as a scaffold on which to place the observed hg H lineages [19] , [20] . This version included a revised version of the hg H sub-tree comprising 1203 sequences in total. As per convention, insertions at np 309.1C(C), 315.1C, 523-524d (aka 522-523d), 16182C, 16183C, 16193.1C(C) and mutation 16519 were not considered for phylogenetic reconstruction [20] . Procrustes-based PCA and Ward Clustering PCA was used to describe and visualise the maternal genetic relationships among the Neolithic cultures investigated, as well as to 37 present-day European and Near Eastern populations ( Fig. 2a ). PCA was performed on the frequency of H sub-hgs taken from the literature ( Supplementary Table S8 ). To minimise statistical noise caused by rare sub-hgs and to allow for data compatibility across published studies, we considered only the following 15 most common H sub-hgs in Europe and the Near East: H*, H1, H1a, H1b, H2, H2a1, H3, H4, H5, H5a, H6, H6a, H7, H8 and H11. PCAs were performed and visualised in R version 2.11.1 (ref. 50 ) using a customised script based on the function prcomp. Ancient hg H individuals were pooled into three different groups based on the numbers of samples available: two for ‘pan-European’ archaeological phenomena/cultures alongside hypothesised geographic origins (LBK, n =9 and BBC, n =7); and a temporally transitional group pooling regional (mostly MNE) cultures (MNE, n =10). Small sample sets such as the Corded Ware ( n =2) and later Bronze Age Unetice ( n =5) were excluded. To test whether the clustering pattern observed in the PCA was significantly supported, we performed a number of statistical tests including Ward clustering, Procrustes analysis and NP-MANOVA (as described below). First, we performed model-based cluster tests to identify the number of clusters via the model with the best support (highest Bayes Information criterion) followed by Ward hierarchical clustering of sub-hg H frequencies using the packages mclust, pvclust (for bootstrap values) and hclust in R, respectively. Procrustes analysis was also performed in R using the package vegan based on PCA scores and geographic coordinates ( Supplementary Table S8 ) and the function protest to calculate the similarity score (100,000 permutations). Summary statistics Population pairwise F ST , Slatkin’s linearised F ST and haplotype diversity were calculated in Arlequin version 3.5 (ref. 51 ). We used jMODELTEST 0.1.1 [52] in order to find the best fitting evolutionary model and, if required, to estimate a discrete γ shape parameter for our 39 non-partitioned mt genomes. Based on the resulting scores for each model (AIC and Bayes Information criterion), we subsequently used the Tamura and Nei model and a γ value of 0.049 for our calculations of population distances in Arlequin. The ancient hg H individuals were pooled into different temporal/cultural groups in order to calculate genetic diversity indices and to test for genetic differentiation ( Table 2 , Supplementary Table S7 ). Multivariate analysis of variance We performed a NP-MANOVA to test whether the temporal grouping of ancient individuals according to archaeological time periods are statistically supported. The NP-MANOVA was performed on a Raup-Crick distance matrix, which was produced from the presence/absence of the 15 hg H sub-hgs used in the PCA. Calculations were performed in PAST version 2.09 with 10,000 permutations per test and post hoc Bonferroni correction to account for multiple comparisons and small sample sizes [53] . We also tested whether the clustering pattern between the ancient and present-day populations observed in the PCA was significantly supported. Bayesian skyride analyses and mutation rate calculation The data set comprised 37 newly sequenced, non-related, ancient mt genomes, five sets of randomly chosen, distinct, present-day hg H mt genomes from Phylotree ( http://www.phylotree.org , mtDNA tree Build 12 (20th July 2011)) and 420 newly available hg H sequences [17] . The Sequences were manually aligned to the revised Cambridge Reference Sequence (rCRS: AC_000021) [54] using the program SeaView [55] . The alignment was partitioned into four subsets, representing the D-loop, the protein-coding regions (1st+2nd codon positions and 3rd codon position) and a concatenation of tRNA and RNA genes. Insertions at nps 309.1C(C), 315.1C, 523-524d (aka 522-523d), 16182C, 16183C, 16193.1C(C) were not considered for phylogenetic reconstruction and position 16519 was removed from the D-loop subset [20] . The best substitution models were selected using ModelGenerator 0.85 (ref. 56 ). by comparison of Bayesian Information Criterion scores: HKY+G for D-loop, TN+G for protein-coding regions and HKY for RNA genes. Considering the short evolutionary timescale being studied (intra-hg), models including a proportion of invariant sites were excluded. A Bayesian skyride analysis [57] was performed using the phylogenetic software BEAST 1.6.1 (ref. 58 ). and calibrated using radiocarbon dates from 18 of the ancient individuals and mean archaeological dates for the remaining individuals. This allowed us to achieve a broad temporal coverage for ~3500 years of the Neolithic period in Central Europe (5500–2000 BC) and to generate the most precise demographic reconstruction of hg H. Results were replicated using independent sets of 100 (1 ×), 200 (3 ×), and 300 (1 ×) mt genomes. A strict molecular clock was used, allowing for a distinct rate in each subset of the alignment. Additional analysis using an uncorrelated log normal relaxed clock to account for potential rate variations could not reject the strict clock assumption. Convergence was checked by sampling from two independent Markov chains. Each MCMC analysis was run for 100,000,000 steps and samples from the two chains were combined, after discarding the first 10% of samples as burn-in. All parameters showed sufficient sampling, indicated by effective sample sizes above 200. Tracer 1.5 was used to produce the skyride plot ( Fig. 1b ) [59] . We carried out a ‘date randomisation test’, to test whether the signal from the radiocarbon dates associated with the ancient sequences was sufficient to calibrate the hg H phylogeny [60] . This test randomises all dates associated with the sequences (including present-day ones) and replicates of the phylogenetic analysis as described above. If the structure and spread of the ancient sequences in the tree were sufficient to calibrate the analysis, the inferred mean rate of the randomised analysis should be significantly different from the rate calculated using the correct association date/sequence. In other words, the 95% HPD of the randomised analysis should not overlap with the mean rate estimated without randomisation. The comparison of estimated rates from the main analysis and from 10 replicates with randomised dates presented in Supplementary Fig. S4 confirms the presence of sufficient signal to calibrate the tree provided by dates from the 37 ancient samples. Accession codes: The complete consensus mt genome sequences have been deposited to NCBI GenBank under accession numbers KC553980 to KC554018 . How to cite this article: Brotherton, P. et al . Neolithic mitochondrial haplogroup H genomes and the genetic origins of Europeans. Nat. Commun. 4:1719 doi: 10.1038/ncomms2656 (2013).